Mechanical work makes important contributions to surface chemistry at steps The effect of mechanical strain on the binding energy of adsorbates to late transition metals is believed to be entirely controlled by electronic factors, with tensile stress inducing stronger binding. Here we show, via computation, that mechanical strain of late transition metals can modify binding at stepped surfaces opposite to well-established trends on flat surfaces. The mechanism driving the trend is mechanical, arising from the relaxation of stored mechanical energy. The mechanical energy change can be larger than, and of opposite sign than, the energy changes due to electronic effects and leads to a violation of trends predicted by the widely accepted electronic ‘d-band’ model. This trend has a direct impact on catalytic activity, which is demonstrated here for methanation, where biaxial tension is predicted to shift the activity of nickel significantly, reaching the peak of the volcano plot and comparable to cobalt and ruthenium. Chemisorption lies at the heart of many important modern technologies and future challenges: catalysts for synthesis, fuel cells for energy production and corrosion for infrastructure sustainability to name a few. Catalysts participate in 90% of all material production [1] , [2] , [3] , playing key roles in the production of commodities such as fertilizer [4] , [5] , [6] , gasoline [1] , [2] , [3] , [7] , [8] , diesel [2] , [3] , [7] , [9] , heating oil [1] , [2] , [3] and pollution scrubbing [2] , [10] , while fuel cells bear the promise of high-efficiency energy production [1] , [11] and corrosion determines the lifetime of infrastructure [12] . With these technologies being of such importance, a fundamental understanding of the underlying mechanisms is essential to design new processes and optimize existing ones. Catalyst design mainly focusses on structure and composition. However, it has been shown both computationally and experimentally that straining of the catalytic surface can affect chemisorption and catalytic activity [13] , [14] , [15] , [16] , [17] , [18] , [19] , [20] , [21] , [22] . In fact, the control of surface strain is a main objective in the design of core/shell nanoparticles, where the lattice mismatch between the core and shell material induces strain on the surface [16] , [17] . The almost-universally held understanding of the effects of strain on the catalytically important late transition metals (LTMs) is that tension strengthens binding [23] . This understanding is supported by an underpinning theory, the ‘d-band model’ that is based on electronic structure. In the d-band model [18] , [19] , [20] , [21] , tensile strain narrows the d-band width, causing an upward shift of the nearly full d-band and thus allows for stronger bonding to adsorbates. All chemisorption processes on LTMs are thus believed to have the same trend with strain [23] . More generally, the effects of strain in other systems are interpreted as electronic in origin [23] , [24] and follow the corresponding trend. Optimal catalytic activity typically involves a balance between competing adsorption and desorption reactions, requiring stronger and weaker binding, respectively [25] . If all chemisorption follows a common trend with strain, then the effects of strain on overall catalytic performance are believed to be relatively small because a given strain cannot cause both stronger and weaker binding of species on a given surface. Here we present extensive computational evidence that the widely held trend of ‘tension strengthens binding’ can be reversed for binding to LTM-stepped surfaces and we show that these trends can be used to tune and enhance catalytic activity. We show that this unexpected trend is entirely mechanical in origin, and is caused by mechanical relaxation that occurs at steps during chemisorption. The mechanical energy change is often larger than the electronic energy change, leading to a reversal, or elimination, of the accepted trend, and thus a violation of the ‘d-band model’, both conceptually and operationally. We further present the mechanics theory that rationalizes the effects and provides the fundamental physical basis for the mechanical effects. The mechanical effect varies with adsorbate and binding site, and thus strain can have a different influence on reactant and product states, leading to large effects on the overall reaction energy. We demonstrate the impact of this mechanical effect on catalytic activity in the specific case of methanation. In this reaction, the mechanical effect completely determines the reactant-binding energy and causes compression to give stronger binding, while both mechanical and electronic effects contribute to the binding of the products with compression giving weaker binding. The difference in trends leads to a strong enhancement of the strain effect, such that an applied strain can move Ni up to the peak activity in the well-established methanation volcano plot, making Ni have the same activity as Ru and Co. With many other important catalytic reactions having controlling processes occurring at surface steps, our results show that mechanical strain can be a valuable design tool for enhancing catalytic activity. Changes in binding energy due to strain We study the chemisorption energies of various adsorbates on various fcc LTM surfaces using the (111) close-packed surface as a model terrace and the (211) surface as a model step. We study three loading cases of applied stress: uniaxial stress normal to the line of the step, σ [−111] , uniaxial stress parallel to the line of the step, σ [01–1] , and biaxial stress in the plane of the surface, σ biax . These applied stresses cause corresponding strains, including Poisson contractions, in the substrate. We unify and discuss the results in terms of the maximum strain component for a given applied stress. We limit our results to a strain range of ±3%. This is within the domain of expected mechanical stability, that is, below strains at which dislocation emission might relax the strains in nanoscale materials. For instance, experiments on nanometre Au pillars show dislocation emission from surface steps at strains above this level [26] and measured shell stresses of greater than 4% have been reported for Cu–Pt/Pt core/shell nanoparticles [16] . Using molecular simulations, we have demonstrated stability of the Cu–Pt/Pt core–shell system with respect to dislocation emission up to at least 4% strain, while others have shown that the energy barriers for dislocation emission from steps in Cu remain significant (several eV) at 3% strain [27] . 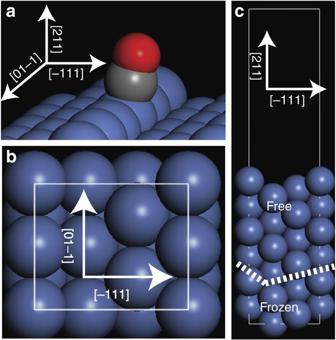Figure 1: Unit cell geometry used to study the fcc(211) surface with a CO molecule bound to the atop site. (a), Model fcc(211) surface with CO molecule bound to the atop position at the step edge; (b), view of slab from the top; and right (c), view of slab from the side, those atoms marked ‘free’ are unconstrained and those marked ‘frozen’ are constrained in the positions determined by continuum elasticity. Figure 1 shows a typical simulation cell used for chemisorption studies of the (211) surface, indicating the two in-plane directions and the CO atop binding configuration. The binding energy E be of some adsorbate X, to some surface S having Miller indices hkl , is defined as Figure 1: Unit cell geometry used to study the fcc(211) surface with a CO molecule bound to the atop site. ( a ), Model fcc(211) surface with CO molecule bound to the atop position at the step edge; ( b ), view of slab from the top; and right ( c ), view of slab from the side, those atoms marked ‘free’ are unconstrained and those marked ‘frozen’ are constrained in the positions determined by continuum elasticity. Full size image We are concerned here with the difference in binding energy with respect to the binding energy at zero applied strain, Thus, comparison issues of absolute energies related to CO bonding are eliminated or minimized [28] , [29] , [30] . We first use the cases of CO* on Ni and Cu to illustrate the scope of new phenomena and new understanding emerging from this work. 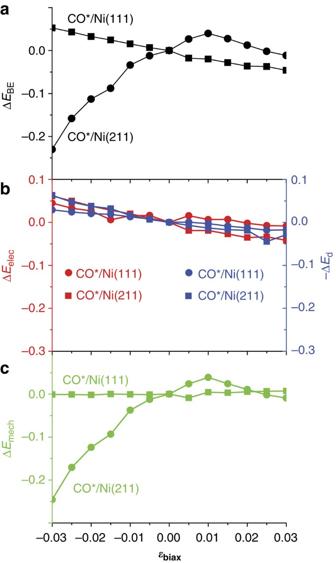Figure 2: Binding energy change versus biaxial strain for CO*/Ni(211) and CO*/Ni(111). (a), Change in binding energy ΔEBEversus strain, showing that the response at the (211) step has increasing binding energy under compressive strain that is opposite from the trend typically found on close-packed (111) surface. (b), Change in electronic contribution to binding, ΔEelec(red), showing the expected increase in binding energy under tensile strain for both (111) and (211), and correlating with the negative of the change in the d-band centre, −ΔEd(blue). (c), Change in mechanical contribution to binding ΔEmech, which is negligible for the (111) terrace but which is large and with compression increasing binding and is responsible for the new trend of increased total binding energy under compressive strain. Vertical axes are in units eV. Figure 2a shows the computed binding energy change due to biaxial stress on CO*/Ni(211) and CO*/Ni(111). The response for Ni(111) shows the expected trend: tensile loading causes stronger binding. In contrast, the response for CO*/Ni(211) is the opposite: compressive loading causes stronger binding, and the magnitude of the effect is comparatively large. Therefore, the chemical response to stress/strain of an adsorbate at a step site can vary from that at a terrace. 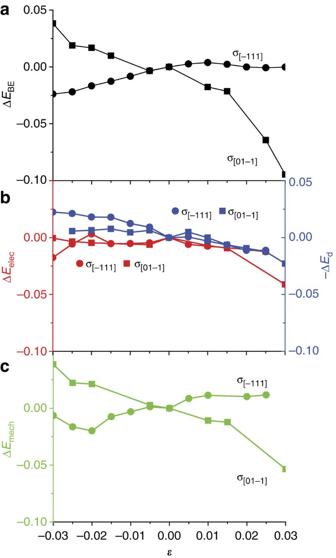Figure 3: Binding energy versus strain for CO*/Cu(211) underσ[−111]andσ[01–1]. (a), Change in binding energy ΔEBEversus strain, showing that compressive stress normal to the step increases the binding energy. (b), Change in electronic contribution to binding, ΔEelec(red), which are small but show the expected increase in binding energy under tensile strain for both (111) and (211), and correlate with the negative of the shift of the d-band centre, −ΔEd(blue), under bothσ[−111]andσ[01–1]loading states. (c), Change in mechanical contribution to binding ΔEmech, which controls the overall energy change (part(a)) for bothσ[−111]andσ[01–1]loading states, withσ[−111]loading causing increased binding under compression. Vertical axes are in units eV. Figure 3a shows the computed binding energy changes for CO*/Cu(211) for various stress states. For the same step site, the binding energy change has two different trends for the two different loading directions. Figures 2a and 3a show clear departures from the expectation that ‘tensile strain causes stronger binding’. This new trend at steps is found for various adsorbates and LTMs ( Supplementary Note 1 ; Supplementary Figs 1–3 ). Even when the net effect of strain on binding at the step is small, the difference in response between step and terrace can be important in many reactions ( Supplementary Note 2 ; Supplementary Figs 3 and 4 ). Generalizing to other adsorbates, Fig. 4 shows the binding energy changes of CO, SH, OH, and NH to Ni(211) and Cu(211) under σ [−111] loading. The trend of stronger adsorbate-binding under compression is found for all these species. The nonvalence binding of a species AX to a surface through A is controlled by A regardless of the X [31] . Thus, the results in Fig. 4 suggest that the new trend will exist for the huge number of catalytic reactions involving binding through C, S, O and N. While we explain the origin of these effects below, the observation that changes in binding due to applied stress are different between terraces and steps and depend on the direction of the applied stress are the first two main results of this paper. Figure 2: Binding energy change versus biaxial strain for CO*/Ni(211) and CO*/Ni(111). ( a ), Change in binding energy Δ E BE versus strain, showing that the response at the (211) step has increasing binding energy under compressive strain that is opposite from the trend typically found on close-packed (111) surface. ( b ), Change in electronic contribution to binding, Δ E elec (red), showing the expected increase in binding energy under tensile strain for both (111) and (211), and correlating with the negative of the change in the d-band centre, −Δ E d (blue). ( c ), Change in mechanical contribution to binding Δ E mech , which is negligible for the (111) terrace but which is large and with compression increasing binding and is responsible for the new trend of increased total binding energy under compressive strain. Vertical axes are in units eV. Full size image Figure 3: Binding energy versus strain for CO*/Cu(211) under σ [−111] and σ [01–1] . ( a ), Change in binding energy Δ E BE versus strain, showing that compressive stress normal to the step increases the binding energy. ( b ), Change in electronic contribution to binding, Δ E elec (red), which are small but show the expected increase in binding energy under tensile strain for both (111) and (211), and correlate with the negative of the shift of the d-band centre, −Δ E d (blue), under both σ [−111] and σ [01–1] loading states. ( c ), Change in mechanical contribution to binding Δ E mech , which controls the overall energy change (part(a)) for both σ [−111] and σ [01–1] loading states, with σ [−111] loading causing increased binding under compression. Vertical axes are in units eV. 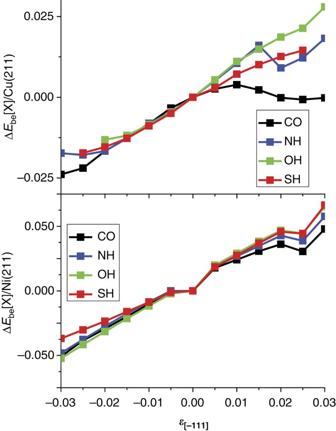Figure 4: Binding energy versus strain for various adsorbates. (a) Cu(211) and (b) Ni(211) under stressσ[−111]normal to the line of the step: CO atop (black), NH bridge (blue), OH bridge (green) and SH bridge (red). All adsorbates show the same trend with stress: compressive stress increases binding energy. Vertical axes are in units eV. Full size image Figure 4: Binding energy versus strain for various adsorbates. ( a ) Cu(211) and ( b ) Ni(211) under stress σ [−111] normal to the line of the step: CO atop (black), NH bridge (blue), OH bridge (green) and SH bridge (red). All adsorbates show the same trend with stress: compressive stress increases binding energy. Vertical axes are in units eV. Full size image Origins of binding energy changes due to strain To interpret the above results, we decompose the binding energy change into two parts: an ‘electronic’ contribution, Δ E elec , due to the totality of surface–adsorbate electronic interactions while holding the substrate ions in their adsorbate-free positions, and a ‘mechanical’ contribution, Δ E mech , associated with the subsequent relaxation of the substrate. This decomposition is shown in Fig. 5a . 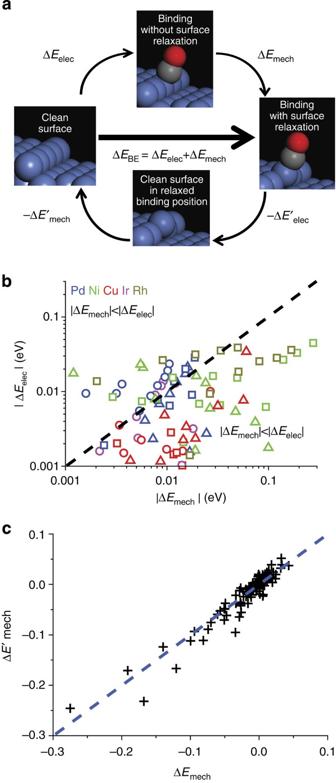Figure 5: Separation and comparison of binding energy changes due to mechanical and electronic contributions. (a) Conceptual separation of the binding energy into an electronic contribution, ΔEelec, due to adsorbate–surface electronic interactions, and a mechanical contribution, ΔEmech, due to structural relaxations upon chemisorption on the strained substrate (distortions exaggerated for emphasis); also shown is the reverse process with corresponding energies ΔE′elecand ΔE′mech, which should have the same trends under loading and with ΔE′mechclearly mechanical in origin. (b) Absolute magnitude of the electronic contribution versus the mechanical contribution, |ΔEelec| versus |ΔEmech|, for CO on various substrates, showing that the mechanical contributions are typically larger than or comparable to the electronic contributions (squares:σbiax; trianglesσ[01–1]; circles:σ[−111]; the color indicates the element as inset). (c) Reverse mechanical contribution ΔE′mechversus forward mechanical contribution ΔEmech, showing that ΔEmech=ΔE′mechholds well (and therefore ΔEelec=ΔE′elec). Dashed line indicates ΔEmech=ΔE′mechand is a guide to the eye. Descriptions of strain state and element in (supplementary Fig 7a). Figure 5a also shows the reverse process: an ‘electronic’ contribution, −Δ E′ elec , due to elimination of the totality of surface–adsorbate electronic interactions while holding the substrate ions fixed in their adsorbate-induced positions, and a ‘mechanical’ contribution, −Δ E′ mech , due to relaxation of the substrate back to the original adsorbate-free structure. The ‘mechanical’ contribution Δ E′ mech is clearly solely due to mechanical effects since the adsorbate is absent in both initial and final states ( Fig. 5a ). With this decomposition, if Δ E′ elec =Δ E elec , and thus Δ E′ mech =Δ E mech , then the electronic contribution to the energy change with strain is independent of the distortions induced by adsorption and the mechanical contribution to the energy change with strain is unquestionably mechanical in nature. As indicated in Fig. 5a , we denote the initial structure under an applied load as ‘undef’ (undeformed by the adsorbate), and the adsorbate-induced structure as ‘def’. The energy contributions are given by the following pair of equations: Figure 5: Separation and comparison of binding energy changes due to mechanical and electronic contributions. ( a ) Conceptual separation of the binding energy into an electronic contribution, Δ E elec , due to adsorbate–surface electronic interactions, and a mechanical contribution, Δ E mech , due to structural relaxations upon chemisorption on the strained substrate (distortions exaggerated for emphasis); also shown is the reverse process with corresponding energies Δ E′ elec and Δ E′ mech , which should have the same trends under loading and with Δ E′ mech clearly mechanical in origin. ( b ) Absolute magnitude of the electronic contribution versus the mechanical contribution, |Δ E elec | versus |Δ E mech |, for CO on various substrates, showing that the mechanical contributions are typically larger than or comparable to the electronic contributions (squares: σ biax ; triangles σ [01–1] ; circles: σ [−111] ; the color indicates the element as inset). ( c ) Reverse mechanical contribution Δ E′ mech versus forward mechanical contribution Δ E mech , showing that Δ E mech =Δ E′ mech holds well (and therefore Δ E elec =Δ E′ elec ). Dashed line indicates Δ E mech =Δ E′ mech and is a guide to the eye. Descriptions of strain state and element in ( supplementary Fig 7a ). Full size image Summing the two gives the total binding energy defined previously, E be = E elec + E mech . We then compute the changes in these contributions as a function of strain as Similar forms apply to Δ E′ elec and Δ E′ mech as given in the Supplementary Note 3 . We note that the energy due to relaxation upon adsorption at zero applied strain is known to be non-negligible [21] , [32] ; however, this energy does not appear in equation (4) when we consider the energy change at finite strain relative to zero strain. We also note that all energies here are computed with density functional theory (DFT), so that the mechanical energy change is associated with the total energy change due to full relaxation of the electrons and ions of the substrate when subjected to the applied strain. The electronic contributions, Δ E elec , for the chemisorption cases of Figs 2a and 3a are shown in Figs 2b and 3b . Also shown is the (negative of) computed d-band centre shifts for the site-projected d-band, which according to the d-band theory should have the same trend as Δ E elec . For both (111) and (211) surfaces, and all loading cases, the electronic contributions show the expected behaviour: tensile stress strengthens binding and correlates with the shift of the d-band centre. The mechanical contributions, Δ E mech , are shown in Figs 2c and 3c . For the close-packed (111) terrace case, Fig. 2c shows that the mechanical energy change is nearly zero and thus the total binding energy change is determined by the electronic contribution and thus follows the expected trend. In distinct contrast, for the Ni(211)-stepped surface, the mechanical contribution is large and opposite to the expected trend: positive for tension and negative for compression. Similarly, Fig. 3c shows that under loading normal to the line of the step, the mechanical contribution for (211) Cu is large and also of the opposite trend: positive for tension and negative for compression. In both (211) cases, the trend of the changes in binding is controlled by the mechanical contribution. Furthermore, Fig. 3c shows that even for the Cu [−110] loading case, where the changes in binding energy follow ‘expected’ trends, the mechanical contribution dominates the electronic contribution. Observation of the ‘expected’ trend therefore does not even mean that the trend is electronic in origin. To reinforce that the mechanical energy change is dominant, Fig. 5b shows the absolute values of Δ E elec, and Δ E mech for CO adsorbates on various strained (211) stepped surfaces. In essentially all cases, the mechanical contribution is comparable to or larger than the electronic contribution. The ratio |Δ E mech |/|Δ E elec | exceeds 10 in 10% of the cases, exceeds 5 in 25% of the cases and has a median value of 1.7 across all 136 cases studied. Moreover, Fig. 5c shows that Δ E′ mech =Δ E mech (and therefore Δ E′ elec =Δ E elec ), demonstrating that the mechanical contribution and mechanical/electronic decomposition are robust. We conclude, in general, that the total binding energy change versus applied stress for stepped surfaces is often dominated by the mechanical contribution, causing overall trends that can often violate the long-standing expectations based on the electronic contribution alone. This is the third main result of this paper. The new trends for the mechanical contribution to adsorbate-binding energy change due to strain can be understood within the framework of mechanics theory. When an adsorbate binds to a surface, under zero applied stress, it causes some deformations in the substrate. These deformations can be characterized by a spatially varying strain tensor with components , and a corresponding stored mechanical energy that is one part of the total binding energy at zero applied strain. When forces or displacements are applied to the substrate material, without an adsorbate, they cause a spatially varying ‘applied’ stress tensor with components in the substrate, and a corresponding stored mechanical energy. When the adsorbate binds to the stressed substrate, there is an additional mechanical interaction energy equal to the work done by the adsorbate-induced displacements against the forces due to the applied stress. If the deformations caused by the adsorbate and the applied stress are both small, so that the material remains in the linear elastic regime, then this mechanical interaction energy is given, in continuum form, by where a summation over the repeated indices i and j is implicit and the integral is over the volume of the system (derivation in Supplementary Note 4 ). The mechanical interaction energy of equation (5) provides a framework for interpreting the results of Figs 2 , 3 , 4 , as follows: because the stresses and strains are tensorial in nature, the mechanical interaction energy depends on the ‘direction’ of the applied stress for a given adsorbate strain; this is consistent with the direction dependence of binding to loading ( Fig. 3c ); on a flat traction-free surface, the stress component perpendicular to the surface is zero. If the adsorbate-induced strain is primarily out-of-plane (for example, lifting up or pushing down of the substrate atoms), then the mechanical interaction energy should be small; this is consistent with all results on terraces ( Fig. 2c and Supplementary Fig. 4 ). At the (211) step, the local stresses near the step tend to follow the applied stress ( Supplementary Note 5 ; Supplementary Fig. 8a ). Therefore, if the corresponding adsorbate-induced strain components are generally positive (stretching) then an applied compressive stress should create a negative mechanical interaction energy, Δ E mech , as found here for most of the step cases under compression ( Figs 2c , 3c and 4 , Supplementary Fig. 3 ); equation (5) shows that Δ E mech is crucially dependent on the strains induced by the adsorbate throughout the substrate volume. Artificially constraining the deformation of the substrate by using small supercells and/or fixed atoms, as carried out in most literature studies, suppresses the mechanical interaction energy (example shown in Supplementary Note 6 , Supplementary Fig. 9 ); this may also account for the absence of stress-driven d-band violations in much of the published literature. If the material mechanical response is nonlinear but reversible, the mechanical interaction energy is more complicated but the essence remains similar to equation (5). Equation (5) is familiar in other chemical contexts, such as the thermodynamic energy p Δ V associated with a point defect of misfit volume Δ V in a matrix under a hydrostatic pressure p [33] , arising in, for example, hydrogen storage in metals and lithium ion batteries. Thus, the existence of the mechanical energy contribution is quite natural and, as shown in Fig. 5b and Supplementary Fig. 7 in the present context of chemical binding versus strain, the mechanical contributions to changes in binding are generally larger than electronic changes. The application of the mechanics theory to rationalize our first three main results is the fourth main result of this paper. Our results suggest a new engineering principle for the control/modulation of catalytic reactions through the application of mechanical strain, whether the strain is because of an applied stress or is induced because of a lattice mismatch, as in pseudomorphic layers and core/shell nanoparticles. We recall that the rate at which a catalyst synthesizes products from reactants is ultimately the result of competing reactions, and that maximum activity is achieved by finding an optimal balance between these competing reactions. If the competing reaction energies scale similarly with strain, then there is strong cancellation of the strain effects. However, if the competing reactions scale differently with strain, as shown here to occur at steps, then there can be a strong enhancement of the strain effects and the possibility of using strain to enhance overall catalytic activity. We now demonstrate this key concept with an explicit example. To predict the effect of mechanical strain on activity, we consider the methanation reaction (CO+3H 2 ↔CH 4 +H 2 O), which has been studied in depth in refs 34 , 35 and highlighted in ref. 25 , in which the activity for unstrained Ni, Rh, Ru, Co and Fe are measured and predicted, as shown in Fig. 6c . The catalytic activity scales with the dissociation energy of the CO molecule, E diss (CO)= E (C+O) −E (CO), with CO on a bridge site of the step and C and O at sites near the step [36] . We have computed the changes in binding and dissociation energies with strain as shown in Fig. 6a,b for Ni. E (CO) exhibits the strong opposite trend (compression increases binding) highlighted in Figs 2 , 3 , 4 , 5 and Supplementary Figs 3 and 5 . Furthermore, Fig. 6a shows the breakdown of E (CO) into mechanical and electronic contributions, and demonstrates that the mechanical contribution completely determines the binding energy change, with nearly zero electronic contribution. In contrast, Fig. 6a shows that the binding energy versus strain for E (C+O) shows the expected trend of tension increasing the binding energy. However, decomposition into mechanical and electronic contributions shows that E (C+O) is a combination of electronic and mechanical contributions. Because the reactant E (CO) and the product E (C+O) follow opposite trends with strain, the dissociation energy E diss (CO)= E (C+O)− E (CO) exhibits a very strong variation with mechanical strain, as shown in Fig. 6b . Following ref 34 , 35 , we use our computed E diss (CO) versus strain to predict the activity of Ni for biaxially strained up to ±3%. As shown in Fig. 6c , we predict that the activity of Ni strained to 3% biaxial tension can reach the peak of the volcano plot; that is, strained Ni can attain the maximum predicted and measured activity. From a chemical perspective for this reaction, the straining of Ni can thus effectively transform Ni into Ru or Co; mechanical strain is thus a new alchemy. The demonstration that opposing trends in chemisorption energy versus strain on the same substrate can have a significant influence on catalytic activity and transform suboptimal materials into peak-performing materials is the fifth main result of this paper. 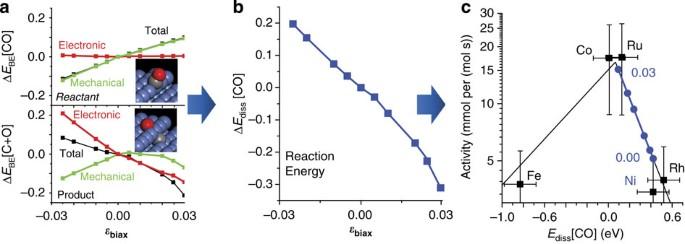Figure 6: Application of mechanical strain to enhance the methanation reaction on Ni. (a) Binding energy changes versus biaxial strain for the reactant CO and product C+O on Ni; compression increases binding of CO and is controlled by the mechanical contribution, while both mechanical and electronic contributions contribute to binding of C+O. (b) Resulting CO dissociation reaction energyEdiss[CO] on Ni, showing a strong variation with strain due to the difference in behaviour between reactant and product shown ina. (c) Methanation activity versusEdiss[CO] (black lines: volcano plot computed in refs34,35; solid squares: experimental/computational results of Anderssonet al. on unstrained Ni, Rh, Ru, Co and Fe; error bars according to ref34; blue circles: current predictions for Ni under biaxial strain using results from 0 to 3 % in steps of 0.5%. Biaxial strain (+3%) in Ni can move the Ni activity up to the peak activity of the volcano plot. Strain can thus make the suboptimal catalyst Ni optimal, and shift the activity of Ni to be equal to the activity of Co or Ru. Figure 6: Application of mechanical strain to enhance the methanation reaction on Ni. ( a ) Binding energy changes versus biaxial strain for the reactant CO and product C+O on Ni; compression increases binding of CO and is controlled by the mechanical contribution, while both mechanical and electronic contributions contribute to binding of C+O. ( b ) Resulting CO dissociation reaction energy E diss [CO] on Ni, showing a strong variation with strain due to the difference in behaviour between reactant and product shown in a . ( c ) Methanation activity versus E diss [CO] (black lines: volcano plot computed in refs 34 , 35 ; solid squares: experimental/computational results of Andersson et al . on unstrained Ni, Rh, Ru, Co and Fe; error bars according to ref 34 ; blue circles: current predictions for Ni under biaxial strain using results from 0 to 3 % in steps of 0.5%. Biaxial strain (+3%) in Ni can move the Ni activity up to the peak activity of the volcano plot. Strain can thus make the suboptimal catalyst Ni optimal, and shift the activity of Ni to be equal to the activity of Co or Ru. Full size image We have shown that the application of mechanical stress can change the binding energy of adsorbates at surface steps of LTMs in an unexpected way—tensile stresses can decrease binding energy and compressive stresses increase binding energy—the opposite of established trends on close-packed surfaces. The new trend is controlled by mechanical interaction energies rather than electronic interaction energies, and is rationalized through a mechanics analysis of the interaction between the adsorbate-induced strains and the applied stress. Most importantly, the existence of this new trend indicates that application of mechanical stress provides new avenues to increase overall catalytic activity for many processes in which the controlling reactions occur at steps. We have demonstrated the impact of this general strategy by showing that methanation on strained Ni is predicted to reach the peak activity of the volcano plot. In total, the results here demonstrate a new scientific phenomenon, the intimate interaction between chemistry and mechanics and the importance of the new phenomenon for enhancing catalytic activity in industrial processes. Density functional theory We use spin-polarized Revised Perdew–Burke–Ernzerhof DFT as implemented in Vienna ab initio simulation package (VASP) [37] , [38] , [39] . A Monkhorst–Pack automatic k-mesh generation scheme was used with 40 subdivisions along each reciprocal lattice vector; the k-mesh was shifted with respect to the origin by 0.5 reciprocal lattice vectors. Owing to the inherent distortions associated with the application of strain, care was taken not to utilize symmetry-based algorithms. A kinetic energy cutoff of 700 eV was used in all calculations [30] . Electronic structure calculations were converged to 1 × 10 −5 eV. Ionic relaxation calculations were converged to 1 × 10 −4 eV. All metals studied (Ni, Cu, Rh, Pd, Ag, Ir, Pt and Au) are fcc. Defining E i as the energy level of the d-band state, E f as the Fermi-level, n d (E i ) as the density-of-states of the d-band at the energy E i , the projected d-band centre E d was computed as the centroid of the d-band, using the same definitions, the projected d-band width W d was calculated as The radius used to determine the projected d-band on an atom was 2.480 Å for Cu and 2.430 Å for Ni. Linear elasticity for strains Material lattice parameters were determined using a conventional fcc cubic unit cell and minimizing the stress tensor. Uniaxial strain and pure shear were applied to determine the c 11 , c 12 and c 44 components of the stiffness tensor. Vicinal fcc(111) surfaces and the stepped fcc(211) surface were studied. A six-layer structure was used, with the bottom two layers frozen in bulk strained configuration, and the top four layers free to relax. The vacuum spacing was ~15 Å. The application of stress to the simulation cell was accomplished by first rotating the stiffness tensor from the conventional fcc cubic cell basis ( m 1 , m 2 , m 3 )=([1,0,0], [0,1,0], [0,0,1]) into the coordinate frame ( e 1 , e 2 , e 3 )=([−1,1,1] /√(3), [0,1,−1]/√(2), [2,1,1]/√(6)) of the DFT unit cell. Within the 6 × 6 matrix representation of the fourth rank stiffness tensor, the rotation was accomplished using the matrix to give the stiffness tensor in the rotated coordinate system as Where The rotated stiffness tensor C (e) was then used to compute the strain corresponding to a desired applied stress using to Hooke’s law, σ = C , and the resulting strain tensor was imposed on the DFT simulation cell. We considered three different applied stresses for (211): (i) uniaxial stress in the [−1,1,1] direction normal to the line of the step, denoted by σ [−111] , (ii) uniaxial stress in the [0,1,−1] direction parallel to the line of the step, denoted by σ [01−1] and (iii) biaxial stress in the plane defined by [−1,1,1] and [0,1,−1] directions, denoted by σ biax . For (111) we consider the established case of biaxial loading. In presenting results, we quote the maximum strain component. How to cite this article: Francis, M. F. et al . Mechanical work makes important contributions to surface chemistry at steps. Nat. Commun. 6:6261 doi: 10.1038/ncomms7261 (2015).